The non-muscle-myosin-II heavy chain Myh9 mediates colitis-induced epithelium injury by restricting Lgr5+ stem cells Lgr5+ stem cells are crucial to gut epithelium homeostasis, and therapies targeting these cells hold promise for treatment of gastrointestinal diseases. Here we report that the non-muscle-myosin-II (NMII) heavy chain Myh9 accumulates at epithelial injury sites in mice distal colon treated with dextran sulphate sodium (DSS). Gut-epithelium-specific Myh9 monoallelic deletion alleviates DSS-induced colonic crypt damage and acute colitis. Consistently, the NMII inhibitor blebbistatin can improve the survival of Lgr5+ stem cells and the growth of Lgr5 organoids. Mechanistically, inhibition of NMII by blebbistatin or Myh9 monoallelic deletion activates Akt through Rac1 and PAK1, which is essential for the survival and pluripotency of Lgr5+ cells. These results establish a critical role of the Myh9-Rac1-PAK1-Akt pathway in the maintenance of Lgr5+ stem cells. As blebbistatin can mitigate DSS-induced colitis and preserve Lgr5+ colonic stem cells in vivo , our findings provide a potential therapeutic intervention of gastrointestinal epithelium injury and degenerative diseases. The gastrointestinal epithelium undergoes rapid self-renewal in adult mammals [1] . Accumulative evidence suggests that there are two types of gut epithelial stem cells: the fast proliferating leucine-rich repeat containing G protein-coupled receptor 5-positive (Lgr5+) cells that maintain intestine and colon homeostasis, and the quiescent Bmi1+ (+4) cells that contribute to intestine regeneration after radiant injury [2] , [3] . These two types of epithelial stem cells can interconvert in the intestinal epithelium [4] . Under physiological conditions, Lgr5+ stem cells actively proliferate and differentiate into all types of cells in the intestinal and colonic epithelium. Several signalling pathways, including Wnt, bone morphogenetic protein (BMP) and Notch, have been demonstrated to regulate the fate of Lgr5+ stem cells [5] . However, the molecular mechanism of how self-renewal and differentiation are balanced in Lgr5+ stem cells remains unclear. Non-muscle-myosin-II (NMII) is a two-headed conventional myosin, which plays key roles in multiple cellular functions, such as mitosis and migration [6] . Its heavy chain has three isoforms in mice, including Myh9, Myh10 and Myh14, among which Myh9 accounts >80% of the total [7] , [8] . Recent studies revealed that dissociation-induced actin-myosin contraction caused the apoptosis of embryonic and induced-pluripotent stem cells [9] , [10] , [11] . However, the detailed mechanism of how NMII regulates stem cell survival remains unclear, and the potential roles of NMII in adult stem cells have not yet been investigated. Feeding mice with dextran sulphate sodium (DSS) polymers in drinking water induces an acute colitis characterized by epithelium damage, bloody diarrhoea, ulceration and granulocyte infiltration, resembling ulcerative colitis in humans [12] , [13] . DSS causes damage to colonic epithelial cells of the basal crypts and affects the integrity of the mucosal barrier. Lgr5+ colonic stem cells are sensitive to DSS treatment and play critical roles in colonic epithelium regeneration [14] , [15] . Therefore, the DSS-induced acute colitis is a good model for investigation of the injury and regeneration of colonic crypts and the functions of Lgr5+ stem cells. In this study, we report that Myh9 is upregulated at epithelial injuries in distal colon treated with DSS, and genetically reducing Myh9 expression alleviates DSS-induced colonic crypt damage. In addition, inhibition of NMII by the small molecule blebbistatin activates Akt through Rac1 and PAK1 and enhances the survival and pluripotency of Lgr5+ stem cells. Finally, blebbistatin also efficiently mitigates DSS-induced colitis and preserves Lgr5+ colonic stem cells in vivo . These results reveal a novel signalling pathway that regulates Lgr5+ stem cell survival and pluripotency, and implicates a potential clinical application of blebbistatin to treat gastrointestinal epithelium injury and degeneration. Myh9 monoallelic deletion ameliorates DSS-induced colitis To search for potential drugs to treat colitis, we established the DSS-induced acute colitis mouse model. After administration of 3% DSS in drinking water for 5 days, most of the mice effectively developed acute colitis. In this process, we noticed an elevated expression of Myh9 in the colonic epithelium ( Fig. 1a ). Immunostaining also confirmed enhanced expression of Myh9 at epithelial injuries, but not the neighbouring epithelium of distal colon ( Fig. 1b ), suggesting that Myh9 is upregulated in DSS-induced colonic epithelium lesions. 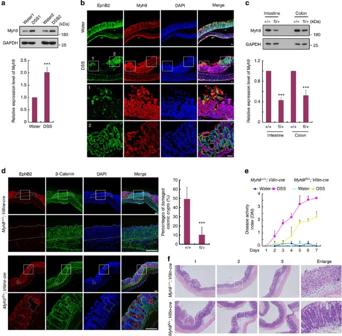Figure 1: Myh9 monoallelic deletion ameliorates epithelial injuries in distal colon treated with DSS. (a) The colonic epithelia were isolated from 8-week-old male mice treated with water or 3% DSS for 5 days followed by 2-day water feeding for immunoblotting with the indicated antibodies. GAPDH served as a loading control. The statistical data represent mean±s.d. (n(the number of mice in each group)=5). (b) Confocal cross-sectioning shows the epithelium injuries in distal colon treated with DSS. Mice treated with 3% DSS for 5 days followed by 2-day water feeding were killed. The distal colon was visualized by immunofluorescence with anti-EphB2 (green) and anti-Myh9 (red). Bottom: enlargements (1: damaged area; 2: normal epithelium). Nuclei were counter-stained with DAPI (blue). A representative data of three independent experiments was shown. Scale bar, 50 μm. (c) Intestinal and colonic epithelia of 8-week-old maleMyh9+/+;Villin-creandMyh9fl/+;Villin-cremice were isolated for immunoblotting with the indicated antibodies. GAPDH served as a loading control. +/+:Myh9+/+;Villin-crefl/+:Myh9fl/+;Villin-creThe statistical data represent mean±s.d. (n=3). (d) Confocal cross-sectioning shows the epithelial injuries in distal colon treated with DSS.Myh9+/+;Villin-creandMyh9fl/+;Villin-cremice were treated with 3% DSS for 5 days followed by 2-day water feeding before being killed. The distal colon was visualized by immunofluorescence with anti-EphB2 (red) and anti-β-catenin (green). The damaged crypts in colonic epithelium are outlined. Bottom: enlargements of the square areas. Scale bar, 100 μm. The statistical analysis of the percentages of damaged colonic crypts in five pairs of mice was shown. The data represent mean±s.d. (n=5). (e) Eight-week-old maleMyh9+/+;Villin-creandMyh9fl/+;Villin-cremice were supplied with water or 3% DSS for 5 days followed by 2-day water feeding. The weight loss, stool consistency and rectal bleeding were daily scored to calculate the disease activity index (DAI). The data represent mean±s.d. (n=5). (f)Myh9+/+;Villin-creandMyh9fl/+;Villin-cremice were treated with 3% DSS for 5 days followed by 2-day water feeding before being killed. Then, paraffin embedded distal colon tissues were stained with haematoxylin and eosin. A representative data of five independent experiments was shown. Wilcoxon’s rank sum test was used fora,candd. Friedman test was used fore. *** indicatesP<0.001. Scale bar, 100 μm. Figure 1: Myh9 monoallelic deletion ameliorates epithelial injuries in distal colon treated with DSS. ( a ) The colonic epithelia were isolated from 8-week-old male mice treated with water or 3% DSS for 5 days followed by 2-day water feeding for immunoblotting with the indicated antibodies. GAPDH served as a loading control. The statistical data represent mean±s.d. ( n (the number of mice in each group)=5). ( b ) Confocal cross-sectioning shows the epithelium injuries in distal colon treated with DSS. Mice treated with 3% DSS for 5 days followed by 2-day water feeding were killed. The distal colon was visualized by immunofluorescence with anti-EphB2 (green) and anti-Myh9 (red). Bottom: enlargements (1: damaged area; 2: normal epithelium). Nuclei were counter-stained with DAPI (blue). A representative data of three independent experiments was shown. Scale bar, 50 μm. ( c ) Intestinal and colonic epithelia of 8-week-old male Myh9 +/+ ; Villin-cre and Myh9 fl/+ ; Villin-cre mice were isolated for immunoblotting with the indicated antibodies. GAPDH served as a loading control. +/+: Myh9 +/+ ; Villin-cre fl/+: Myh9 fl/+ ; Villin-cre The statistical data represent mean±s.d. ( n =3). ( d ) Confocal cross-sectioning shows the epithelial injuries in distal colon treated with DSS. Myh9 +/+ ; Villin-cre and Myh9 fl/+ ; Villin-cre mice were treated with 3% DSS for 5 days followed by 2-day water feeding before being killed. The distal colon was visualized by immunofluorescence with anti-EphB2 (red) and anti-β-catenin (green). The damaged crypts in colonic epithelium are outlined. Bottom: enlargements of the square areas. Scale bar, 100 μm. The statistical analysis of the percentages of damaged colonic crypts in five pairs of mice was shown. The data represent mean±s.d. ( n =5). ( e ) Eight-week-old male Myh9 +/+ ; Villin-cre and Myh9 fl/+ ; Villin-cre mice were supplied with water or 3% DSS for 5 days followed by 2-day water feeding. The weight loss, stool consistency and rectal bleeding were daily scored to calculate the disease activity index (DAI). The data represent mean±s.d. ( n =5). ( f ) Myh9 +/+ ; Villin-cre and Myh9 fl/+ ; Villin-cre mice were treated with 3% DSS for 5 days followed by 2-day water feeding before being killed. Then, paraffin embedded distal colon tissues were stained with haematoxylin and eosin. A representative data of five independent experiments was shown. Wilcoxon’s rank sum test was used for a , c and d . Friedman test was used for e . *** indicates P< 0.001. Scale bar, 100 μm. Full size image To investigate the pathological significance of Myh9 upregulation at epithelial injuries in the distal colon, we generated gut epithelium tissue-specific Myh9 -knockout mice. Genotyping and examination of Myh9 mRNA and protein levels in intestinal and colonic epithelium confirmed the knockout of one allele of Myh9 in Myh9 fl/+ ; Villin-cre mice ( Fig. 1c and Supplementary Fig. 1 ). However, we did not obtain the complete Myh9 -knockout mouse. It could be due to the early expression of Villin-Cre in the visceral endoderm of E6.5 embryos [16] , and Myh9 ablation leads to severe defects in the visceral endoderm of E6.5 embryos [17] . Myh9 fl/+ ; Villin-cre mice exhibited no obvious abnormality in intestinal or colonic epithelium homeostasis ( Supplementary Fig. 2 ). When exposed to 3% DSS, however, only mild colonic epithelium injury was observed in Myh9 fl/+ ; Villin-cre mice, which was in contrast to severe colonic damage in Myh9 +/+ ; Villin-cre mice ( Fig. 1d ). These data suggest that Myh9 may be involved in DSS-induced colonic epithelium injuries. As colonic epithelium injuries are critical for colitis initiation [13] , [14] , [15] , we then accessed whether Myh9 monoallelic loss could alleviate DSS-induced acute colitis. The disease activity index (DAI) has been commonly used to evaluate the grade and extent of acute colitis [18] . The DAI score ranges from 0 to 4, representing the sum of scores for weight loss, stool consistency and rectal bleeding, divided by three. As shown in Fig. 1e , DSS treatment led to severe colitis as shown by high DAI scores, while the water feeding group did not exhibit any colitis symptoms. Myh9 monoallelic deletion led to significantly decreased DAI scores following DSS treatment ( Fig. 1e ). Consistently, milder crypt damage ( Fig. 1f ), better proliferation status ( Supplementary Fig. 3a ) and less apoptosis ( Supplementary Fig. 3b ) were observed in distal colon epithelium of Myh9 fl/+ ; Villin-cre mice following DSS treatment, compared with Myh9 +/+ ; Villin-cre mice. These data suggest that Myh9 plays an important role in DSS-induced colitis process. Dissociation-induced Myh9 expression restricts crypt growth To further investigate the functions of Myh9 in crypt damages, we mechanically dissociated small intestinal and colonic crypts, embedded them in Matrigel and performed in vitro culture according to the previous report [19] . We found that Myh9 mRNA increased markedly in both small intestinal and colonic crypts immediately after dissociation ( Fig. 2a ). In addition, small intestinal and colonic crypts isolated from Myh9 fl/+ ; Villin-cre mice survived better than those from Myh9 +/+ ; Villin-cre mice ( Fig. 2b ). Knockdown of Myh9 expression using adenovirus-based shRNA promoted the survival of isolated crypts ( Supplementary Fig. 4a,b ). These results together suggest that dissociation-induced Myh9 expression restricts crypt survival. 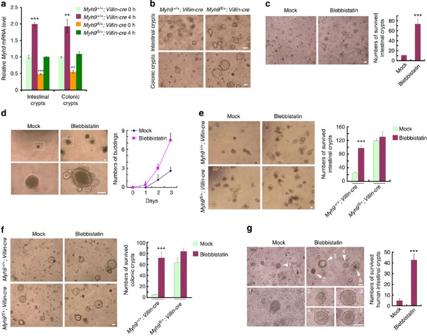Figure 2: Dissociation-induced Myh9 expression restricts crypt survival and growth. (a) Intestinal and colonic crypts dissociated from 8-week-old maleMyh9+/+;Villin-creandMyh9fl/+;Villin-cremice were embedded in Matrigel for the indicated time and harvested to examineMyh9expression using quantitative RT-PCR.Gapdhwas used as an internal control. (b) One hundred intestinal and colonic crypts isolated fromMyh9+/+;Villin-creandMyh9fl/+;Villin-cremice were embedded in Matrigel and cultured in the presence of EGF, Noggin and R-spondin1 (ENR) for 24 h. A representative data of three independent experiments was shown. (c) One hundred isolated mouse intestinal crypts were embedded in Matrigel and cultured in the presence of ENR for 24 h. DMSO (mock) or blebbistatin (10 μM) was added in the culture medium. (d) Isolated crypts were cultured for 3 days in the ENR culture medium in the absence or presence of blebbistatin (10 μM). The organoid buddings were quantified, and the data represent mean±s.d. (n=5). (e) Isolated intestinal crypts were cultured in the presence of ENR, together with DMSO (mock) or 10 μM blebbistatin for 2 days. (f) Isolated colonic crypts were cultured in the presence of ENR, together with DMSO (mock) or 10 μM blebbistatin for 36 h. (g) One hundred human intestinal crypts isolated from normal intestinal tissues were embedded in Matrigel and cultured in the presence of ENR, together with DMSO (mock) or 10 μM blebbistatin for 36 h. The statistical analyses of survived crypt numbers were shown, and the data represent mean±s.d. (n=3). Kruskal-Wallis’ H test was used fora,eandf. Student’st-test was used forc,dandg. *** indicatesP<0.001. ** indicatesP<0.01. Scale bar, 50 μm. Figure 2: Dissociation-induced Myh9 expression restricts crypt survival and growth. ( a ) Intestinal and colonic crypts dissociated from 8-week-old male Myh9 +/+ ; Villin-cre and Myh9 fl/+ ; Villin-cre mice were embedded in Matrigel for the indicated time and harvested to examine Myh9 expression using quantitative RT-PCR. Gapdh was used as an internal control. ( b ) One hundred intestinal and colonic crypts isolated from Myh9 +/+ ; Villin-cre and Myh9 fl/+ ; Villin-cre mice were embedded in Matrigel and cultured in the presence of EGF, Noggin and R-spondin1 (ENR) for 24 h. A representative data of three independent experiments was shown. ( c ) One hundred isolated mouse intestinal crypts were embedded in Matrigel and cultured in the presence of ENR for 24 h. DMSO (mock) or blebbistatin (10 μM) was added in the culture medium. ( d ) Isolated crypts were cultured for 3 days in the ENR culture medium in the absence or presence of blebbistatin (10 μM). The organoid buddings were quantified, and the data represent mean±s.d. ( n =5). ( e ) Isolated intestinal crypts were cultured in the presence of ENR, together with DMSO (mock) or 10 μM blebbistatin for 2 days. ( f ) Isolated colonic crypts were cultured in the presence of ENR, together with DMSO (mock) or 10 μM blebbistatin for 36 h. ( g ) One hundred human intestinal crypts isolated from normal intestinal tissues were embedded in Matrigel and cultured in the presence of ENR, together with DMSO (mock) or 10 μM blebbistatin for 36 h. The statistical analyses of survived crypt numbers were shown, and the data represent mean±s.d. ( n =3). Kruskal-Wallis’ H test was used for a , e and f . Student’s t -test was used for c , d and g . *** indicates P< 0.001. ** indicates P< 0.01. Scale bar, 50 μm. Full size image Consistently, blebbistatin (1,2,3,3a-tetrahydro-3a-hydroxy-6-methyl-1-phenyl-4H- pyrrolo[2,3-b]quinolin-4-one), a reversible inhibitor of NMII heavy chain [20] , [21] , could significantly benefit the survival of mouse intestinal crypts ( Fig. 2c ). Typical fields taken at day 3 showed that crypt cultures treated with blebbistatin formed larger organoids than untreated ones, and more budding crypts were observed ( Fig. 2d ), indicating that blebbistatin facilitates the growth of Lgr5 organoids. The promoting effect of blebbistatin was not observed in the crypts from Myh9 fl/+ ; Villin-cre mice as these crypts already had a high survival rate ( Fig. 2e,f ), consistent with the idea that blebbistatin mainly works through inhibiting Myh9. Blebbistatin also markedly promoted the survival of human intestinal crypts and colonic crypts ( Fig. 2g and Supplementary Fig. 4c ). Myh9 regulates the survival and pluripotency of Lgr5+ cells Lgr5+ stem cells are critical for gut homeostasis [2] , and these stem cells are ablated in distal colon following DSS treatment [14] . To address whether Myh9 regulates Lgr5+ stem cell survival, we employed Lgr5-EGFP-IRES-creERT2 mice to analyse Myh9 expression in Lgr5+ stem cells upon DSS treatment. Administration of 3% DSS in drinking water for 2 days led to an elevation of the total Myh9-high cell number (from 31%=29.17+1.75 to 45%=42.7+2.28) as well as in the Lgr5-GFP-positive population (from 28.6%=1.75/(1.75+4.37) to 49.5%=2.28/(2.28+2.32)) ( Fig. 3a ). In accordance, DSS treatment also decreased the expression of the Lgr5+ stem cell marker genes Lgr5 and Sox9 , and Myh9 monoallelic deletion efficiently rescued the reduction ( Fig. 3b ). These results further demonstrate the restricting function of Myh9 in Lgr5+ stem cell survival in DSS-treated distal colon. 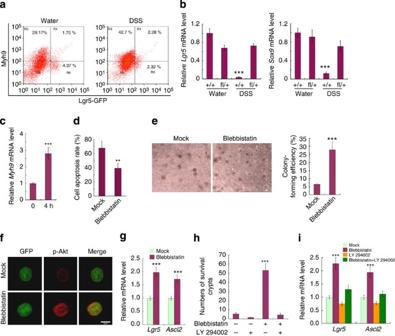Figure 3: Myh9 controls the survival and pluripotency of Lgr5+ stem cells in an Akt-dependent manner. (a) Eight-week-old maleLgr5-EGFP-IRES-creERT2mice were supplied with water or 3% DSS for 2 days before being killed. The distal colon crypt cells were isolated and subjected to anti-Myh9 FACS. (b) Mice were treated with 1.5% DSS for 5 days followed by 2-day water feeding before being killed. The distal colon crypts were harvested to examineLgr5andSox9expression using qRT-PCR. +/+:Myh9+/+;Villin-crefl/+:Myh9fl/+;Villin-cre.(c) Single Lgr5-GFPhi cells isolated from the intestinal crypts ofLgr5-EGFP-IRES-creERT2mice were embedded in Matrigel for the indicated time before harvesting to examineMyh9expression using qRT-PCR. (d) Cultured single Lgr5-GFPhi cells were with treated DMSO (mock) or 10 μM blebbistatin for 6 h. Then, the cells were stained with Propidium Iodide and subjected to FACS. (e) Five hundred single Lgr5-GFPhi cells isolated from the intestinal crypts ofLgr5-EGFP-IRES-creERT2mice were treated with DMSO or 10 μM blebbistatin for 2 days, then blebbistatin was withdrawn, and cultures were maintained to day 7 and photographed. Scale bar, 50 μm. The colony-forming efficiencies were calculated and the statistical analysis was shown. (f) Single Lgr5-GFPhi cells were treated with DMSO or 10 μM blebbistatin for 12 h and subjected to anti-phospho-Akt immunoflourescence. Scale bar, 5 μm. (g) Lgr5-GFP+ organoids were treated with DMSO or blebbistatin (10 μM) for 12 h. The Lgr5-GFPhi cells were isolated by FACS and harvested to examineLgr5andAscl2expression using qRT-PCR. (h) Isolated crypts were treated with 10 μM blebbistatin and/or 25 μM LY294002 for 24 h. Crypt number was accounted. (i) Lgr5-GFP+ organoids were treated with 10 μM blebbistatin and/or 25 μM LY294002 for 12 h. The Lgr5-GFPhi cells were isolated by FACS to examineLgr5andAscl2expression with qRT-PCR. For qRT-PCR,Gapdhwas used as an internal control. The statistical data represent mean±s.d. (n=3).aandfare representative of three independent experiments. Kruskal-Wallis’ H test was used forb. Student’st-test was used forc,d,eandg. ANOVA test was used forhandi. ***IndicatesP<0.001. **IndicatesP<0.01. Figure 3: Myh9 controls the survival and pluripotency of Lgr5+ stem cells in an Akt-dependent manner. ( a ) Eight-week-old male Lgr5-EGFP-IRES-creERT2 mice were supplied with water or 3% DSS for 2 days before being killed. The distal colon crypt cells were isolated and subjected to anti-Myh9 FACS. ( b ) Mice were treated with 1.5% DSS for 5 days followed by 2-day water feeding before being killed. The distal colon crypts were harvested to examine Lgr5 and Sox9 expression using qRT-PCR. +/+: Myh9 +/+ ; Villin-cre fl/+: Myh9 fl/+ ; Villin-cre. ( c ) Single Lgr5-GFPhi cells isolated from the intestinal crypts of Lgr5-EGFP-IRES-creERT2 mice were embedded in Matrigel for the indicated time before harvesting to examine Myh9 expression using qRT-PCR. ( d ) Cultured single Lgr5-GFPhi cells were with treated DMSO (mock) or 10 μM blebbistatin for 6 h. Then, the cells were stained with Propidium Iodide and subjected to FACS. ( e ) Five hundred single Lgr5-GFPhi cells isolated from the intestinal crypts of Lgr5-EGFP-IRES-creERT2 mice were treated with DMSO or 10 μM blebbistatin for 2 days, then blebbistatin was withdrawn, and cultures were maintained to day 7 and photographed. Scale bar, 50 μm. The colony-forming efficiencies were calculated and the statistical analysis was shown. ( f ) Single Lgr5-GFPhi cells were treated with DMSO or 10 μM blebbistatin for 12 h and subjected to anti-phospho-Akt immunoflourescence. Scale bar, 5 μm. ( g ) Lgr5-GFP+ organoids were treated with DMSO or blebbistatin (10 μM) for 12 h. The Lgr5-GFPhi cells were isolated by FACS and harvested to examine Lgr5 and Ascl2 expression using qRT-PCR. ( h ) Isolated crypts were treated with 10 μM blebbistatin and/or 25 μM LY294002 for 24 h. Crypt number was accounted. ( i ) Lgr5-GFP+ organoids were treated with 10 μM blebbistatin and/or 25 μM LY294002 for 12 h. The Lgr5-GFPhi cells were isolated by FACS to examine Lgr5 and Ascl2 expression with qRT-PCR. For qRT-PCR, Gapdh was used as an internal control. The statistical data represent mean±s.d. ( n =3). a and f are representative of three independent experiments. Kruskal-Wallis’ H test was used for b . Student’s t -test was used for c , d , e and g . ANOVA test was used for h and i . ***Indicates P< 0.001. **Indicates P< 0.01. Full size image Then, we sorted single Lgr5-GFPhi cells from Lgr5-EGFP-IRES-creERT2 mouse intestine and cultured them in Matrigel under the condition described previously [19] . We observed that Myh9 mRNA significantly increased in Lgr5+ stem cells immediately after dissociation ( Fig. 3c ). Remarkably, blebbistatin inhibited the dissociation-induced apoptosis of single Lgr5+ stem cells ( Fig. 3d ) and markedly enhanced their colony-forming efficiency ( Fig. 3e ) and their proliferation ( Supplementary Fig. 5 ), indicating that Myh9 inhibition promotes the survival of Lgr5+ stem cells. Cell survival is tightly controlled by phosphoinositide-3-phosphate kinase (PI3K)-Akt signalling [22] . It has been shown that Akt activity, as shown by Akt phosphorylation, is critical for the expansion of intestinal crypts and epithelial stem cells [23] , [24] , [25] . Therefore, we hypothesized that blebbistatin might activate Akt in Lgr5+ stem cells. To test this, sorted single Lgr5-GFPhi cells were embedded in Matrigel, treated with blebbistatin for 12 h and then stained for phosphorylated Akt. The data from both immunofluorescence and FACS revealed that blebbistatin enhanced Akt phosphorylation in Lgr5+ stem cells ( Fig. 3f and Supplementary Fig. 6 ). The PI3K-Akt signal pathway has also been shown to support the pluripotency of embryonic stem cells [26] , [27] . Furthermore, Akt has been suggested to promote self-renewal of +4 intestinal stem cells through the activation of Wnt-β-catenin signalling [25] . As blebbistatin can activate Akt, we then attempted to address whether blebbistatin is able to improve the pluripotency of Lgr5+ intestinal stem cells. As shown in Fig. 3g , blebbistatin stimulated the expressions of the pluripotency marker genes Lgr5 and Ascl2 in Lgr5+ intestinal stem cells [2] , [28] . To further support the notion that blebbistatin promotes the survival and pluripotency of Lgr5+ stem cells via Akt activation, we examined whether the PI3K-specific inhibitor LY294002, which can block Akt activation [29] , could attenuate the effects of blebbistatin. The data in Fig. 3h demonstrated that LY294002 efficiently abolished the promoting effect of blebbistatin on crypt survival. In accordance, blebbistatin could not enhance the expression levels of Lgr5 or Ascl2 in the presence of LY294002, compared with blebbistatin alone ( Fig. 3i ). Furthermore, the Akt inhibitor MK2206 [30] decreased the survival of Myh9 fl/+ ; Villin-cre crypts ( Supplementary Fig. 7 ). These results together suggest that Akt activity is essential for Myh9 inhibition to promote the survival and pluripotency of Lgr5+ stem cells. Myh9-mediated actin-myosin contraction has been suggested to be involved in dissociation-induced apoptosis of embryonic and induced-pluripotent stem cells [9] , [10] , [11] . We then tested whether disruption of actin filament polymerization could also improve the survival of isolated crypts. Unlike blebbistatin, neither cytochalasin D that prevents actin polymerization [31] nor swinholide A that severs actin filaments [32] could promote crypt survival ( Supplementary Fig. 8a,b ), indicating that actin-myosin contraction is not involved in the inhibitory effect of Myh9 on crypt survival. Consistently, inhibition of myosin light chain phosphorylation by the MLC kinase inhibitor ML-7 had no effect on crypt survival ( Supplementary Fig. 8c ). Rac1 and PAK1 mediate Akt activation by blebbistatin We then explored the molecular mechanism how blebbistatin activates Akt. As it was technically difficult to obtain enough Lgr5+ stem cells for biochemical analyses, we searched several colon carcinoma cell lines (LS174T, SW480, HCT116 and HT29) to analyse the effect of blebbistatin on Akt activity. However, Akt activity in these cells was not affected by blebbistatin treatment. By screening more cell lines, we found that NIH3T3 cells were sensitive to blebbistatin in Akt activation ( Fig. 4a ). Basal Akt phosphorylation in NIH3T3 cells decreased over time under normal growth condition ( Fig. 4b ). In contrast, blebbistatin treatment induced Akt activation within 30 min and maintained its high phosphorylation level up to 12 h. Consistently, reducing Myh9 expression in intestinal crypts also resulted in elevated Akt phosphorylation ( Fig. 4c ), in agreement with the note that Myh9 is the major target of blebbistatin to promote crypt survival. 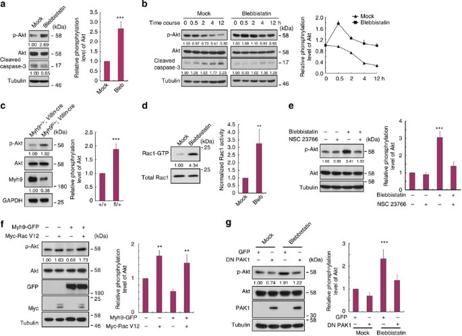Figure 4: Inhibition of NMII heavy chain activates Akt through Rac1 and PAK1. (a) NIH3T3 cells were treated with DMSO (mock) or 10 μM blebbistatin for 12 h and harvested for immunoblotting with the indicated antibodies. The numbers underneath each gel indicate the relative band densities after normalized to controls. (b) NIH3T3 cells were treated with DMSO (mock) or 10 μM blebbistatin for the indicated time, and harvested for immunoblotting. (c) Intestinal crypts ofMyh9+/+;Villin-creandMyh9fl/+;Villin-cremice were isolated for immunoblotting with the indicated antibodies. GAPDH served as a loading control. +/+:Myh9+/+;Villin-crefl/+:Myh9fl/+;Villin-cre. (d) The activation states of endogenous Rac1 in NIH3T3 cells treated with DMSO (mock) or 10 μM blebbistatin for 12 h were detected by the effector pull-down assay. Cell lysates were incubated with the agarose-immobilized GST-PAK1(RBD), and the co-precipitates were subjected to anti-Rac1 immunoblotting. (e) NIH3T3 cells treated with the indicated chemicals for 12 h were harvested for immunoblotting. (f) NIH3T3 cells transfected with Myh9-GFP and Myc-Rac(V12) were harvested for immunoblotting. (g) NIH3T3 cells infected with lentiviral GFP or DN PAK1(N-SP) were treated with DMSO (mock) or 10 μM blebbistatin for 12 h, and harvested for immunoblotting. Tubulin served as a loading control. The statistical data represent mean±s.d. (n=3). Wilcoxon’s rank sum test was used fora,candd. Friedman test was used forb. Kruskal-Wallis’ H test was used fore–g. ***IndicatesP<0.001. **IndicatesP<0.01. Figure 4: Inhibition of NMII heavy chain activates Akt through Rac1 and PAK1. ( a ) NIH3T3 cells were treated with DMSO (mock) or 10 μM blebbistatin for 12 h and harvested for immunoblotting with the indicated antibodies. The numbers underneath each gel indicate the relative band densities after normalized to controls. ( b ) NIH3T3 cells were treated with DMSO (mock) or 10 μM blebbistatin for the indicated time, and harvested for immunoblotting. ( c ) Intestinal crypts of Myh9 +/+ ; Villin-cre and Myh9 fl/+ ; Villin-cre mice were isolated for immunoblotting with the indicated antibodies. GAPDH served as a loading control. +/+: Myh9 +/+ ; Villin-cre fl/+: Myh9 fl/+ ; Villin-cre . ( d ) The activation states of endogenous Rac1 in NIH3T3 cells treated with DMSO (mock) or 10 μM blebbistatin for 12 h were detected by the effector pull-down assay. Cell lysates were incubated with the agarose-immobilized GST-PAK1(RBD), and the co-precipitates were subjected to anti-Rac1 immunoblotting. ( e ) NIH3T3 cells treated with the indicated chemicals for 12 h were harvested for immunoblotting. ( f ) NIH3T3 cells transfected with Myh9-GFP and Myc-Rac(V12) were harvested for immunoblotting. ( g ) NIH3T3 cells infected with lentiviral GFP or DN PAK1(N-SP) were treated with DMSO (mock) or 10 μM blebbistatin for 12 h, and harvested for immunoblotting. Tubulin served as a loading control. The statistical data represent mean±s.d. ( n =3). Wilcoxon’s rank sum test was used for a , c and d . Friedman test was used for b . Kruskal-Wallis’ H test was used for e – g . ***Indicates P< 0.001. **Indicates P< 0.01. Full size image We found that blebbistatin induced activation of Rac1 ( Fig. 4d ), a GTPase involved in a diverse set of cellular processes including proliferation, apoptosis, migration and invasion. Recent studies have demonstrated that Rac1 can activate Akt [33] , [34] , and Rac1 plays a critical role in Lgr5+ stem cells expansion [35] . To test whether Rac1 mediates Akt activation by blebbistatin, using NSC23766, a specific Rac1 inhibitor [36] , we observed that inhibition of Rac1 abolished blebbistatin-induced Akt phosphorylation ( Fig. 4e ). Furthermore, overexpression of Myh9 decreased endogenous Akt activity, which could be rescued by Rac1(V12), a constitutively active form of Rac1 [37] ( Fig. 4f ). These data together suggest that Rac1 mediates blebbistatin-induced Akt activation. It has been reported that Rac1 stimulates Akt activity through a kinase-independent scaffolding function of PAK1 [34] . We then assessed the possible involvement of PAK1 in blebbistatin-induced Akt activation. PAK1(N-SP) (the N-terminal fragment of PAK1, 1-205aa, with the substitution of Ser76 with proline), a dominant-negative mutant disrupting the scaffolding function of PAK1 [34] , effectively abolished the effect of blebbistatin to activate Akt ( Fig. 4g ). Taken together, these data indicate that inhibition of Myh9 by blebbistatin activates Akt in a manner dependent on Rac1 and PAK1. To assess the significance of the Myh9-Rac1-Akt axis in Lgr5+ intestinal stem cells, we first confirmed that blebbistatin could activate Rac1 in cultured intestinal organoids ( Fig. 5a ). We then assessed whether Rac1 inactivation could attenuate blebbistatin-induced phosphorylation of Akt in single Lgr5-GFPhi cells. Immunostaining results revealed that the Rac1 inhibitor NSC23766 effectively impaired the activity of blebbistatin to activate Akt in Lgr5+ stem cells ( Fig. 5b ). Consistently, NSC23766 abolished the promoting effect of blebbistatin or Myh9 monoallelic loss on the survival of isolated crypts ( Fig. 5c,d ) and the growth of Lgr5 organoids ( Fig. 5e ). In addition, the accelerated growth of Lgr5 organoids induced by blebbistatin treatment or Myh9 deficiency was blocked by PAK1(N-SP) ( Fig. 5f,g ). These data together indicate that Myh9 inhibition by blebbistatin activates Akt in Lgr5+ intestinal stem cells through the Rac1-PAK1 axis. 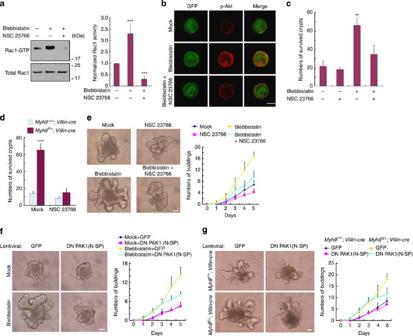Figure 5: The Rac1-PAK1-Akt axis is essential for Myh9 inhibition to promote the survival and pluripotency of Lgr5+ stem cells. (a) The activation states of endogenous Rac1 in cultured intestinal organoids treated with 10 μM blebbistatin and 100 μM NSC23766 for 12 h were detected by the effector pull-down assay. Cell lysates were incubated with the agarose-immobilized GST-PAK1(RBD), and the co-precipitates were subjected to anti-Rac1 immunoblotting. (b) Single Lgr5-GFPhi cells embedded in Matrigel were cultured in the medium containing ENR, Wnt3a, DMSO (mock), 10 μM blebbistatin and 100 μM NSC23766 for 12 h and subjected to immunoflourescence analysis with an anti-phospho-Akt antibody. A representative data of three independent experiments was shown. Scale bar, 5 μm. (c) Isolated intestinal crypts were cultured in the ENR medium together with 10 μM blebbistatin and 100 μM NSC23766 for 24 h and counted. (d) Crypts isolated fromMyh9+/+;Villin-creandMyh9fl/+;Villin-cremice were cultured in the ENR medium together with 10 μM blebbistatin and 100 μM NSC23766 for 24 h and counted. (e) Isolated intestinal crypts were cultured for 5 days in the ENR medium together with 10 μM blebbistatin and 100 μM NSC23766. Scale bar, 50 μm. (f) Isolated intestinal crypts were infected with lentivirus expressing GFP or PAK1(N-SP), and cultured for 5 days in the ENR medium with or without blebbistatin (10 μM). (g) Crypts isolated fromMyh9+/+;Villin-creandMyh9fl/+;Villin-cremice were infected with lentivirus expressing GFP or PAK1(N-SP), and cultured for 5 days in the ENR medium with or without blebbistatin (10 μM). The organoid buddings were quantified, and the data represent mean±s.d. (n=5). The statistical results ina,canddrepresent mean±s.d. (n=3). Kruskal-Wallis’ H test was used foraandd. ANOVA test was used forc. Friedman test was used fore–g. ***IndicatesP<0.001. **IndicatesP<0.01. Scale bar, 50 μm. Figure 5: The Rac1-PAK1-Akt axis is essential for Myh9 inhibition to promote the survival and pluripotency of Lgr5+ stem cells. ( a ) The activation states of endogenous Rac1 in cultured intestinal organoids treated with 10 μM blebbistatin and 100 μM NSC23766 for 12 h were detected by the effector pull-down assay. Cell lysates were incubated with the agarose-immobilized GST-PAK1(RBD), and the co-precipitates were subjected to anti-Rac1 immunoblotting. ( b ) Single Lgr5-GFPhi cells embedded in Matrigel were cultured in the medium containing ENR, Wnt3a, DMSO (mock), 10 μM blebbistatin and 100 μM NSC23766 for 12 h and subjected to immunoflourescence analysis with an anti-phospho-Akt antibody. A representative data of three independent experiments was shown. Scale bar, 5 μm. ( c ) Isolated intestinal crypts were cultured in the ENR medium together with 10 μM blebbistatin and 100 μM NSC23766 for 24 h and counted. ( d ) Crypts isolated from Myh9 +/+ ; Villin-cre and Myh9 fl/+ ; Villin-cre mice were cultured in the ENR medium together with 10 μM blebbistatin and 100 μM NSC23766 for 24 h and counted. ( e ) Isolated intestinal crypts were cultured for 5 days in the ENR medium together with 10 μM blebbistatin and 100 μM NSC23766. Scale bar, 50 μm. ( f ) Isolated intestinal crypts were infected with lentivirus expressing GFP or PAK1(N-SP), and cultured for 5 days in the ENR medium with or without blebbistatin (10 μM). ( g ) Crypts isolated from Myh9 +/+ ; Villin-cre and Myh9 fl/+ ; Villin-cre mice were infected with lentivirus expressing GFP or PAK1(N-SP), and cultured for 5 days in the ENR medium with or without blebbistatin (10 μM). The organoid buddings were quantified, and the data represent mean±s.d. ( n =5). The statistical results in a , c and d represent mean±s.d. ( n =3). Kruskal-Wallis’ H test was used for a and d . ANOVA test was used for c . Friedman test was used for e – g . ***Indicates P< 0.001. **Indicates P< 0.01. Scale bar, 50 μm. Full size image BMP signalling induces Myh9 expression We next set out to determine how Myh9 accumulated at epithelial injuries after DSS treatment. Interestingly, we noticed that BMP signalling was highly activated at epithelial injuries, as indicated by the increased phospho-Smad1/5 ( Fig. 6a ). To test whether BMP signalling participates in dissociation-induced Myh9 expression, the cultured Lgr5 organoids were dissociated from Matrigel and passaged. Indeed, the passaging-induced dissociation process elevated the Myh9 mRNA level significantly ( Fig. 6b ), which coincided with the increase of the BMP target Id1 expression ( Supplementary Fig. 9 ). Withdrawal of the BMP inhibitor Noggin from the culture medium after organoid passaging further increased Myh9 mRNA expression ( Fig. 6b ), consistent with upregulation of both Myh9 mRNA and protein by BMP treatment in Lgr5 organoids ( Fig. 6c,d ). Altogether, our data suggest that DSS-induced epithelium injuries and the organoid dissociation process elevate BMP signalling, which can stimulate Myh9 expression. 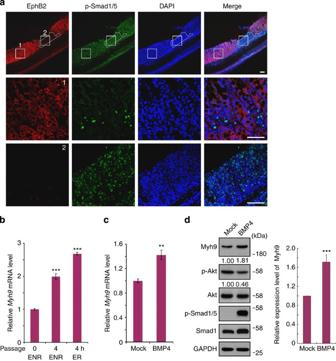Figure 6: BMP signalling mediates dissociation-induced Myh9 upregulation. (a) Confocal cross-sectioning shows the epithelial injuries in distal colon treated with DSS. Eight-week-old male mice supplied with 3% DSS for 5 days followed by 2-day water feeding were killed. The distal colon was examined by immunofluorescence with anti-EphB2 (red) and anti-p-Smad1/5 (green). The injury regions on colonic epithelium are outlined. Bottom: enlargements (1: normal epithelium; 2: damaged area). A representative data of three independent experiments was shown. Scale bar, 100 μm. (b) Intestinal organoids cultured in the ENR medium were dissociated from Matrigel and passaged in the medium containing ENR or ER for 4 h. Then, the organoids were harvested to examineMyh9expression using quantitative RT-PCR.Gapdhwas used as an internal control. (c) Intestinal organoids cultured in the ER medium were treated with 10 ng ml−1BMP4 for 4 h and harvested to examineMyh9expression using quantitative RT-PCR.Gapdhwas used as an internal control. (d) Intestinal organoids cultured in the ER medium were treated with 10 ng ml−1BMP4 for 12 h and harvested for immunoblotting. GAPDH served as a loading control. The statistical data represent mean±s.d. (n=3). ANOVA test was used forb. Student’st-test was used forc. Wilcoxon’s rank sum test was used ford. ***IndicatesP<0.001. **IndicatesP<0.01. Figure 6: BMP signalling mediates dissociation-induced Myh9 upregulation. ( a ) Confocal cross-sectioning shows the epithelial injuries in distal colon treated with DSS. Eight-week-old male mice supplied with 3% DSS for 5 days followed by 2-day water feeding were killed. The distal colon was examined by immunofluorescence with anti-EphB2 (red) and anti-p-Smad1/5 (green). The injury regions on colonic epithelium are outlined. Bottom: enlargements (1: normal epithelium; 2: damaged area). A representative data of three independent experiments was shown. Scale bar, 100 μm. ( b ) Intestinal organoids cultured in the ENR medium were dissociated from Matrigel and passaged in the medium containing ENR or ER for 4 h. Then, the organoids were harvested to examine Myh9 expression using quantitative RT-PCR. Gapdh was used as an internal control. ( c ) Intestinal organoids cultured in the ER medium were treated with 10 ng ml −1 BMP4 for 4 h and harvested to examine Myh9 expression using quantitative RT-PCR. Gapdh was used as an internal control. ( d ) Intestinal organoids cultured in the ER medium were treated with 10 ng ml −1 BMP4 for 12 h and harvested for immunoblotting. GAPDH served as a loading control. The statistical data represent mean±s.d. ( n =3). ANOVA test was used for b . Student’s t -test was used for c . Wilcoxon’s rank sum test was used for d . ***Indicates P< 0.001. **Indicates P< 0.01. Full size image Blebbistatin alleviates colitis and preserves Lgr5+ cells As blebbistatin could promote the survival and pluripotency of Lgr5+ stem cells and improve crypt cultures, we then tested whether blebbistatin had beneficial effect on DSS-induced epithelium injury and colitis in vivo . As shown in Fig. 7a , DSS treatment led to severe colitis as shown by high DAI scores, while the control group did not exhibit any colitis symptoms. Daily intraperitoneal injection of blebbistatin significantly decreased the DSS-caused DAI scores and also protected the structure of distal crypts ( Fig. 7b ). These data suggest that blebbistatin can efficiently alleviate DSS-induced colitis in mice. 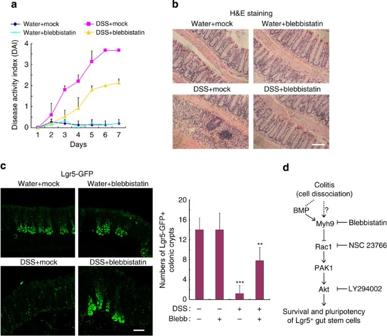Figure 7: Blebbistatin alleviates DSS-induced colitis and preserves Lgr5+ colonic stem cells. (a) Eight-week-old male mice supplied with water or 3% DSS for 5 days followed by 2-day water feeding were daily injected with mock or blebbistatin. The weight loss, stool consistency and rectal bleeding were daily scored to calculate the disease activity index (DAI). The data represent mean±s.d. (n=5). (b) Mice supplied with water or 3% DSS for 5 days followed by 2-day water feeding were daily injected with mock or blebbistatin. Then, paraffin embedded distal colon tissues were stained with haematoxylin and eosin. A representative data of five independent experiments was shown. (c) Eight-week-old maleLgr5-EGFP-IRES-creERT2mice fed with water or 1.5% DSS for 5 days followed by 2-day water feeding were daily injected with mock or blebbistatin, and Lgr5+ colonic stem cells in distal colon were examined by confocal cross-sectioning. The statistical analysis of the numbers of Lgr5-GFP+ colonic crypts in five independent experiments was shown. The data represent mean±s.d. Friedman test was used fora. Kruskal-Wallis’ H test was used forc. *** indicatesP<0.001. ** indicatesP<0.01. Scale bar, 100 μm. (d) Working model of the Myh9-Rac1-PAK1-Akt signalling pathway to mediate colitis-induced damage on Lgr5+ stem cells. Figure 7: Blebbistatin alleviates DSS-induced colitis and preserves Lgr5+ colonic stem cells. ( a ) Eight-week-old male mice supplied with water or 3% DSS for 5 days followed by 2-day water feeding were daily injected with mock or blebbistatin. The weight loss, stool consistency and rectal bleeding were daily scored to calculate the disease activity index (DAI). The data represent mean±s.d. ( n =5). ( b ) Mice supplied with water or 3% DSS for 5 days followed by 2-day water feeding were daily injected with mock or blebbistatin. Then, paraffin embedded distal colon tissues were stained with haematoxylin and eosin. A representative data of five independent experiments was shown. ( c ) Eight-week-old male Lgr5-EGFP-IRES-creERT2 mice fed with water or 1.5% DSS for 5 days followed by 2-day water feeding were daily injected with mock or blebbistatin, and Lgr5+ colonic stem cells in distal colon were examined by confocal cross-sectioning. The statistical analysis of the numbers of Lgr5-GFP+ colonic crypts in five independent experiments was shown. The data represent mean±s.d. Friedman test was used for a . Kruskal-Wallis’ H test was used for c . *** indicates P< 0.001. ** indicates P< 0.01. Scale bar, 100 μm. ( d ) Working model of the Myh9-Rac1-PAK1-Akt signalling pathway to mediate colitis-induced damage on Lgr5+ stem cells. Full size image To test whether the beneficial effect of blebbistatin on colonic epithelium is related to the improved maintenance of Lgr5+ stem cells, we examined Lgr5+ colonic stem cells in Lgr5-EGFP-IRES-creERT2 mice. Administration of 1.5% DSS in mice drinking water for 5 days led to the ablation of GFP-positive Lgr5+ stem cells in the distal colon, and blebbistatin injection efficiently prevented their loss ( Fig. 7c ). Notably, the mice treated with blebbistatin showed equivalent CD45+ immune cell infiltration into the epithelium and the lamina propria ( Supplementary Fig. 10 ), indicating that blebbistatin protected Lgr5+ stem cells independently of anti-inflammation. These data together suggest that blebbistatin alleviates DSS-induced colitis by preserving Lgr5+ colonic stem cells. Colitis and other intestine degenerative diseases are common human disorders, but the clinical interventions are limited as the pathological mechanisms are not very clear. Using the DSS-induced mouse acute colitis model, we observed an elevated expression of non-muscle-myosin-II heavy chain Myh9 at the epithelial injuries. Genetically reducing the expression of Myh9 or inhibiting its activity by blebbistatin ameliorated colonic epithelium injury and acute colitis. Mechanistically, interference of Myh9 activity enhanced the survival and pluripotency of Lgr5+ stem cells via the Rac1-PAK1-Akt signalling pathway ( Fig. 7d ). DSS-induced acute colitis is a widely employed model to study colitis, which is thought to be provoked by inflammation [13] , [38] , [39] . However, recent studies suggest that damage of colonic stem cells could be a major cause [13] , [14] , [15] . In addition, disruption of epithelial cell contacts could be important in the pathological process as the loss of tight junctions of colonic epithelial cells was observed in DSS-induced colitis [40] , [41] , [42] . We observed that Myh9 was upregulated in DSS-induced colonic epithelial injuries and in Lgr5+ stem cells on dissociation. BMP signalling, which was activated in the injuries and dissociated organoids, partially contributed to Myh9 upregulation. Activation of BMP signalling in the DSS-induced injuries could also have a negative impact on Lgr5+ stem cells. However, inhibition of BMP signalling with Noggin could not completely abolish the dissociation-induced Myh9 expression, indicating other pathways should participate in this process. The mechanism how the epithelial cell dissociation regulates Myh9 expression in vivo needs further investigation. We demonstrated that depletion or inhibition of Myh9 greatly improved the survival and pluripotency maintenance of Lgr5+ gut stem cells, indicating that the restricting effect of NMII is not limited to embryonic or induced-pluripotent stem cells. Previous studies showed that actomyosin hyperactivation led to dissociation-induced apoptosis of embryonic and induced-pluripotent stem cells [9] , [10] , [11] . Although it is still controversial whether this type of cell death belongs to anoikis, the consensus was that the excessive actin-myosin contraction caused by loss of E-cadherin-dependent intercellular contact is critical for dissociation-induced death of embryonic or induced-pluripotent stem cells. However, a different mechanism must be involved in Lgr5+ stem cells as none of the actin disruption drugs we have tested could improve the survival of dissociated crypts. Together with the observation that inhibition of myosin light chain phosphorylation by ML-7 had no effect on Lgr5+ stem cell survival, our data indicate that Myh9-mediated Lgr5+ stem cell death is independent of dissociation-induced actin-myosin contraction. This idea is consistent with a recent report showing that Myh9 could function as a novel tumour suppressor of squamous cell carcinomas through activating p53 independent of F-actin polymerization [43] . It is currently unclear why different mechanisms are employed in the negative effect of Myh9 on different stem/pluripotent cells. A possibility could be the differences of culture conditions for different types of stem cells, as Lgr5+ stem cells and Lgr5 organoids were cultured in the 3-D Matrigel system, while previous reported embryonic and induced-pluripotent stem cells were cultured in 2-D dishes. Of note, blebbistatin-induced Akt activation was observed only in Lgr5+ intestinal stem cells and NIH3T3 cells among the cell lines we have examined, further showing the cell-type-specific regulation of Akt activity by Myh9. Lgr5+ stem cells play dominant roles in gut epithelium homeostasis and regeneration [2] , [14] , [15] , [44] , [45] . Our data for the first time demonstrated that Myh9 restricts the survival and pluripotency of Lgr5+ stem cells through inhibiting Akt in DSS-induced colitis. Akt activation has been demonstrated to be important to maintain self-renewal of embryonic stem cells and Bmi1+ intestinal stem cells [25] , [26] , [27] . It has been suggested that Akt activates Wnt/β-catenin signalling, which plays the dominant role in Lgr5+ stem cell self-renewal [23] , [46] . Here we demonstrated the important role of the Myh9-Rac1-PAK1-Akt signalling pathway in maintenance of Lgr5+ stem cells. In summary, our in vivo data demonstrated that inhibition of NMII heavy chain by blebbistatin could preserve Lgr5+ colonic stem cells and alleviate DSS-induced colitis, implicating its potential clinical application in the treatment of gastrointestinal epithelium injury and degenerative disease in humans. Our findings also extend the understanding of the signalling pathways controlling Lgr5+ stem cell self-renewal and offer new insights into the roles of NMII heavy chain in adult stem cells. In addition, we showed that blebbistatin greatly improved the Lgr5 organoid cultures, which can be employed to establish an efficient and cost-effective method to maintain Lgr5+ stem cells in vitro . Reagents Blebbistatin and NSC23766 were purchased from Calbiochem, Matrigel from BD Biosciences, recombinant mouse Noggin, recombinant human BMP4 and recombinant human R-Spondin1 from R&D systems, recombinant mouse Wnt-3A from Millipore, Jagged-1 peptide from AnaSpec, MK2206 from Selleckchem, Cytochalasin D and Swinholide A from Biomol, recombinant mouse EGF, Advanced DMEM/F12, TrypLE, Penicillin/Streptomycin, GlutaMAX-I, N2 and B27 from Invitrogen, and N-Acetylcysteine, BSA, DAPI, EDTA, Propidium Iodide, ML-7 and LY 294002 from Sigma. Mice, human tissues and cell line Lgr5-EGFP-ires-creERT2 mice [2] and Villin-cre mice were obtained from the Jackson Laboratory. Myh9 fl/fl mouse sperms were obtained from MMRRC. Myh9 fl/+ ; Villin-cre mice were generated by in vitro fertilization. All animal studies were performed in accordance with the relevant guidelines and regulations and with the approval of the Institutional Animal Care and Use Committee of Tsinghua University. Fresh normal human intestine and colon tissues were obtained immediately after surgery. The epithelium was separated mechanically from fat and other components, followed by isolation of human intestinal or colonic crypts. All experiments were performed in accordance with the relevant guidelines and regulations and with the approval of the Ethics Committee guideline of Peking University Third Hospital. NIH3T3 was obtained from ATCC and maintained in DMEM medium supplemented with 10% FBS (Hyclone) in a 37 °C humidified incubator containing 5% CO 2 . Intestinal crypt isolation, single Lgr5-GFPhi cells purification and culture Mouse intestine was isolated from 8-week-old male mice, cut longitudinally and washed twice with cold PBS. Villi were carefully scraped off with operating scalpel. The remaining part was cut into small pieces (5 mm) and incubated in 10 mM EDTA in PBS for 40 min on ice. After removal of EDTA, the small pieces were vigorously suspended using a 10-ml pipette with cold PBS. The supernatant, which enriched in crypts, was passed through a 70-μm cell strainer (BD) and centrifuged at 600 r.p.m. for 3 min. The pure crypts obtained were used for culture or single Lgr5-GFPhi cell purification. To purify single Lgr5-GFPhi cells, isolated intestinal crypts were treated with TrypLE (Invitrogen) for 30 min, and then syringed using a 1.2-mm needle to obtain a single cell-enriched population. After passing through a 40-μm cell strainer (BD), Lgr5-GFPhi cells were sorted using FACS (BD FACSAria II). Isolated crypts or single Lgr5-GFPhi cells were embedded in Matrigel, followed by seeding on a 48-well plate (50 μl Matrigel per well). After polymerization of Matrigel, crypt culture medium (Advanced DMEM/F12 supplemented with Penicillin/Streptomycin, GlutaMAX-I, N2, B27 and N-acetylcysteine) containing indicated growth factors (50 ng ml −1 EGF, 100 ng ml −1 Noggin and 500 ng ml −1 R-spondin1) was overlaid. In single Lgr5-GFPhi cells culture, 1 mM Jagged-1 peptide was added in Matrigel and 100 ng ml −1 Wnt3a was included in the culture medium. The entire medium was changed every 2 days. Colonic epithelium/crypt isolation Colon from 8-week-old male mice was cut longitudinally and washed twice with cold PBS to remove fetal material. Then, small pieces (5 mm) of colon were incubated in 10 mM EDTA in PBS for 40 min on ice, followed by vigorously suspended using a 10-ml pipette with cold PBS. The supernatant enriched in colonic epithelia was passed through a 70-μm cell strainer (BD) and centrifuged at 600 r.p.m. for 3 min. The collected colonic epithelia were subjected to immunoblot or FACS. If colonic crypts were required, the colonic epithelia isolated were further incubated in TrypLE for 10 min to separate the crypts from the surface epithelial cells. DSS-induced colitis Acute colitis was induced by feeding 8-week-old male C57BL/6 mice with 3% DSS (MP Biomedicals) dissolved in drinking water for 5 days (days 1–5). Intraperitoneal injection of mock or blebbistatin (20 mg kg −1 ) was employed daily. At Day 7 after the start of DSS administration, the mice were killed, and the distal colon was isolated for immunostaining or haematoxylin and eosin staining. For detection of Lgr5+ stem cells in distal colon during colitis, 8-week-old male Lgr5-EGFP-IRES-creERT2 mice were treated with 1.5% DSS for 5 days followed by 2-day water feeding. Then the distal colon was visualized by immunofluorescence. Immunostaining Intestine or distal colon was isolated, fixed with 4% formaldehyde solution and embedded in 4% low-melting-point agarose (Invitrogen). The sections were prepared with vibrating blade microtome (HM650, Microm) and permeabilized with 0.2% Triton X-100 in PBS for 1 h. Isolated Lgr5 organoids or single Lgr5-GFPhi cells were fixed for 1 h with 4% paraformaldehyde at room temperature and permeabilized for 20 min with 0.2% Triton X-100 and blocked for 1 h in 5% BSA. After incubation overnight at 4 °C with the primary antibody, the secondary antibody was added for 1 h at room temperature. The following antibodies were used for immunostaining: α-β-catenin (Santa Cruz, 1:200), α-CD45 (BD Biosciences, 1:100), α-EphB2 (R&D systems, 1:100), α-Myh9 (Proteintech Group, 1:100), α-p-Akt (Ser473) (Cell Signaling, 1:100), α-p-Smad1/5 (Cell Signaling, 1:100), fluorescein isothiocyanate (FITC)-conjugated α-mouse IgG and α-rabbit IgG (Jackson ImmunoResearch, 1:200) and tetramethylrhodamine β-isothiocyanate (TRITC)-conjugated α-mouse IgG and α-rabbit IgG (Jackson ImmunoResearch, 1:200). Confocal laser scanning was done on a Zeiss LSM 710 NLO Laser Scanning Microscope and FACS was done on a BD FACSCalibur system. Immunohistochemistry Tissues were fixed with 4% formalin and embedded in paraffin. Sections were deparaffinized in isopropanol and graded alcohols, followed by antigen retrieval, and endogenous peroxidase quenched by H 2 O 2 . Sections were then blocked with normal goat serum for 30 min, and incubated overnight at 4 °C with a Ki67 antibody (Abcam, 1:200). The secondary biotinylated anti-rabbit antibody (Invitrogen, 1:5000) was added for 30 min, followed by detection with streptavidin-HRP (Invitrogen, 1:500) and DAB+ chromogen (Invitrogen) according to the manufacturer’s recommendations. Slides were counterstained with Mayer’s haematoxylin, dehydrated and mounted with Eukitt. Tunel assay Cell death was assessed by TdT-mediated dUTP nick end labelling (TUNEL) of formalin-fixed paraffin-embedded slides of the respective genotypes using the TUNEL cell death detection kit (Roche). Immunoblotting The assays were performed as previously described [47] . The following antibodies were used for immunoblotting: α-Akt (Cell Signaling, 1:2,000), α-Cleaved caspase-3 (Cell Signaling, 1:1,000), α-GAPDH (Santa Cruz, 1:2,000), α-GFP (Santa Cruz, 1:1,000), α-MLC (Abcam, 1:1,000), α-Myc (Santa Cruz, 1:1,000), α-Myh9 (Proteintech Group, 1:2,000), α-PAK1 (Cell Signaling, 1:1,000), α-p-Akt (Ser473) (Cell Signaling, 1:2,000), α-p-MLC (Cell Signaling, 1:1,000), α-p-Smad1/5 (Cell Signaling, 1:2,000), α-Rac1 (BD Biosciences, 1:1,000), α-Smad1 (Cell Signaling, 1:2,000), α-Tubulin (Santa Cruz, 1:1,000) and ECL HRP-conjugated α-mouse IgG and α-rabbit IgG (GE Healthcare, 1:10,000). The experiments were repeated for at least three times, and representative data were shown. The band intensity was quantified with BandScan 5.0. The signal density of phosphorylated proteins was normalized to the corresponding unphosphorylated proteins. The full immunoblots were provided in Supplementary Information ( Supplementary Fig. 11 ). RNA interference Ad-NS shRNA and Ad- Myh9 shRNA were generated with BLOCK-iT Adenoviral RNAi Expression System (Invitrogen). The target sequences were Ad-NS shRNA (5′-CTACACAAATCAGCGATTT-3′) and Ad- Myh9 shRNA (5′-GGATCAATGTGACCGACTTCA-3′). Lentiviral expression The coding sequences of GFP and PAK1(N-SP) were cloned into pENTR1A plasmid, and LR clonase reactions (Invitrogen) were carried out to place them into the p2k7neo lentiviral backbone [48] . The viral supernatants were used to infect isolated crypts. Quantitative RT-PCR (qRT-PCR) Total RNA was extracted with RNeasy Mini Kit (Qiagen) and cDNA was synthesized with Revertra Ace (Toyobo). A Mx3000p Quantitative PCR system (Stratagene) was employed to perform qRT-PCR. Taqman gene expression assays (Applied Biosystems) were used to detect gene expressions in single Lgr5-GFPhi cells. The assay IDs were Ascl2 (Mm01268891_g1), Gapdh (Mm99999915_g1) and Lgr5 (Mm00438890_m1). EvaGreen dye (Biotium)-based qRT-PCR was performed to detect gene expressions in crypts. The primers were Myh9 (5′-GTGAGAAGGAGACAAAGGCG-3′ and 5′-GACTTCTCCAGCTCGTGGAC-3′), Id1 (5′-ATCGCATCTTGTGTCGCTGAG-3′ and 5′-AGTCTCTGGAGGCTGAAAGGT-3′), Lgr5 (5′-CGGGACCTTGAAGATTTCCT-3′ and 5′-GATTCGGATCAGCCAGCTAC-3′), Sox9 (5′-GCCAGATGGACCCACCAGTAT-3′ and 5′-TCCAAACAGGCAGGGAGATTC-3′) and Gapdh (5′-AAGAAGGTGGTGAAGCAG-3′ and 5′-TCATACCAGGAAATGAGC-3′). Statistical analysis We employed Student’s t -test or ANOVA test to analyse the parametric experimental results. In nonparametric data analysis (histology scores, immunoblots and DAI scores), we employed Wilcoxon’s rank sum test for two-group treatments, Kruskal-Wallis’ H test for multi-group treatments and Friedman test for DAI score analysis along the time. Significant differences were noted with asterisks. How to cite this article: Zhao, B. et al. The non-muscle-myosin-II heavy chain Myh9 mediates colitis-induced epithelium injury by restricting Lgr5+ stem cells. Nat. Commun. 6:7166 doi: 10.1038/ncomms8166 (2015).